Phylogenomic analyses uncover origin and spread of theWolbachiapandemic Of all obligate intracellular bacteria, Wolbachia is probably the most common. In general, Wolbachia are either widespread, opportunistic reproductive parasites of arthropods or essential mutualists in a single group of filarial nematodes, including many species of medical significance. To date, a robust phylogenetic backbone of Wolbachia is lacking and consequently, many Wolbachia -related phenomena cannot be discussed in a broader evolutionary context. Here we present the first comprehensive phylogenomic analysis of Wolbachia supergroup relationships based on new whole-genome-shotgun data. Our results suggest that Wolbachia has switched between its two major host groups at least twice. The ability of some arthropod-infecting Wolbachia to universally infect and to adapt to a broad range of hosts quickly is restricted to a single monophyletic lineage (containing supergroups A and B). Thus, the currently observable pandemic has likely a single evolutionary origin and is unique within the radiation of Wolbachia strains. Like all members of the order Rickettsiales (Alphaproteobacteria), Wolbachia are obligate intracellular symbionts. Main evolutionary Wolbachia lineages are termed ‘supergroups’ [1] and differ markedly in their host distribution and biology. Supergroup A and B Wolbachia strains are found in many groups of terrestrial arthropods, making it one of the most common endosymbionts worldwide. An estimated 40% of all species are infected [2] . In many arthropod hosts, Wolbachia enhance their spread by inducing reproductive alterations such as cytoplasmic incompatibility (CI), parthenogenesis, male-killing and feminization [3] . Although Wolbachia is generally transmitted vertically (from mother to offspring), regular horizontal transmissions between arthropod hosts as well as recurrent gains and losses are evident from a lack of co-cladogenesis of Wolbachia with its hosts [4] , [5] . In stark contrast, Wolbachia of supergroups C and D are found exclusively in some filarial nematodes and their long-lasting intimate association has led to various mutual dependencies [6] . Other distinct Wolbachia strain groups are known only from a small number of hosts: supergroup E is found in springtails (Hexapoda, Collembola), supergroup H in termites (Hexapoda, Isoptera) and further, so far unclassified strains were detected in Ctenocephalides felis (Hexapoda, Siphonaptera), Dipetalonema gracile (Nematoda, Filarioidea), Bryobia sp. (Arachnida, Acari) and Cordylochernes scorpioides (Arachnida, Pseudoscorpiones) [7] , [8] , [9] , [10] , [11] , [12] . The nature of the symbiosis in all of these cases is only superficially understood. Interestingly, supergroup F Wolbachia may infect both arthropods and nematodes, and strains of this supergroup may act as a mutualist and can induce CI [13] , [14] , [15] . Although found in many higher ranked arthropod taxa (for example, insect orders), supergroup F Wolbachia are generally rare [11] . Given the diverging lifestyles of Wolbachia supergroups, the question arises whether Wolbachia from arthropods and nematodes represent distinct, monophyletic evolutionary lineages and, if so, which phylogenetic position can be attributed to supergroup F that is not constrained to a single host group. An intriguing hypothesis suggests that this group is a basal branching lineage that might represent Wolbachia ’s ancestral lifestyle [16] . While phylogenetic analyses of Wolbachia strains based on a single or a few genes usually enable correct supergroup assignments, relationships between supergroups remain poorly resolved and consequently, partially conflicting phylogenetic hypotheses were proposed [11] , [17] , [18] , [19] , [20] . Furthermore, these data sets are especially prone to artefacts caused by recombination between Wolbachia strains [21] . Owing to the fact that hitherto, whole-genome data from supergroups other than A, B, C and D are lacking, phylogenomic analyses (albeit providing well-resolved trees) were restricted to a limited sampling of Wolbachia strains [16] , [22] . In addition, a large evolutionary distance to its closest relatives has hampered an unequivocal rooting of the Wolbachia tree [23] . However, a well-resolved rooted tree is needed to interpret the direction of major lifestyle transitions in Wolbachia ’s evolutionary history. In the present study, we aim to address the major challenges in reconstructing Wolbachia ’s evolutionary history by enhancing taxon and gene sampling. To this end, we created new whole-genome-shotgun (WGS) data of so far unsampled supergroup E from the springtail Folsomia candida , supergroup H from the termite Zootermopsis nevadensis and supergroup F from the solitary bee Osmia caerulescens. A data set of 90 carefully selected single-copy orthologues from these data and from already published Wolbachia genomes (supergroups A, B, C and D) were used for phylogenomic analyses. We integrated various phylogenetic approaches as well as measures to identify and subsequently reduce systematic biases. We consequently present a robust and well-supported phylogenetic hypothesis for the evolution of Wolbachia strains. Our findings indicate that the ubiquitous Wolbachia supergroups A and B belong to a single, monophyletic lineage and consequently, the ability to adapt to a large range of taxonomically and physiologically diverse hosts has a single origin in that lineage. Furthermore, the Wolbachia strains that are obligate mutualists of nematodes are a paraphyletic assemblage, suggesting that host switches from arthopods to nematodes (or back) occurred at least twice in the evolutionary history of Wolbachia . 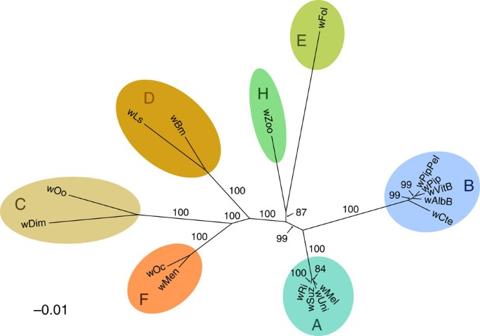Figure 1: Unrooted phylogram showing relationships between investigatedWolbachiastrains. The phylogram was inferred with RAxML from a nucleotide supermatrix including 69,677 base positions. Numbers on clades correspond to bootstrap values in percent from 1,000 replicates. Supergroup affiliations are given in coloured letters. Leaf labels correspond toWolbachiastrain names. Scale bar corresponds to inferred evolutionary changes. Analysis of the same matrix with MrBayes resulted in identical topology with maximal statistical support for all splits. Reconstructing Wolbachia’s evolutionary history To reconstruct Wolbachia supergroup relationships via a phylogenomic pipeline, we utilized available genomic sequences of Wolbachia supergroups A, B, C and D as well as supergroup F Wolbachia sequences originating from a Strepsiptera genome project ( Table 1 ). In addition, we performed WGS sequencing of four arthropod hosts carrying distinct Wolbachia strains so far not represented by genomic data ( Table 1 ). BLAST searches in the corresponding assemblies allowed us to identify most of the 90 loci to be employed for phylogenetic analyses from wOc (87/90), wFol (82/90) and wCte (78/90). For wZoo and wMen, only 19 and 38 loci were recovered, respectively. Preliminary supergroup assignment with multilocus sequence typing (MLST) loci that were extracted from the assemblies showed that wOc and wMen clustered within arthropod and nematode supergroup F strains, and that wFol represents a distinct lineage of the Wolbachia radiation ( Supplementary Fig. 1 ). Unexpectedly and in contrast to previously published results [24] , wCte from the present study fell within supergroup B, suggesting that C. felis populations differ in their endosymbiont composition. Table 1 Origin of sequence data used in this study. Full size table In the single-gene alignments used for subsequent analyses, no evidence for intragenic recombination or nucleotide substitution saturation was detected. The resulting masked supermatrices were composed of 21 taxa and 69,677 and 23,262 characters for nucleotides and amino acids, respectively. Ingroup relationships estimated from all data sets and analyses ( Fig. 1 ; Supplementary Figs 2–5 ) resulted in the same, highly supported topology with the exception of the placement of supergroup H. All supergroups represented by >1 strain were recovered as monophyletic, with the ubiquitous arthropod-infecting Wolbachia A and B being reciprocally monophyletic. The nematode-infecting supergroups (C and D) form a monophyletic group with supergroup F, in which C and F are sister taxa. Only the placement of supergroup H is ambiguous. A sister group relationship with E was not recovered in all analyses ( Supplementary Figs 2–5 ). Figure 1: Unrooted phylogram showing relationships between investigated Wolbachia strains. The phylogram was inferred with RAxML from a nucleotide supermatrix including 69,677 base positions. Numbers on clades correspond to bootstrap values in percent from 1,000 replicates. Supergroup affiliations are given in coloured letters. Leaf labels correspond to Wolbachia strain names. Scale bar corresponds to inferred evolutionary changes. Analysis of the same matrix with MrBayes resulted in identical topology with maximal statistical support for all splits. Full size image The analyses including outgroups Ehrlichia ssp. and Anaplama ssp. yielded identical topologies, again receiving almost maximal support for all nodes ( Fig. 2 ; Supplementary Figs 6–17 ). Once more, the placement of supergroup H was not consistent across analyses and data sets. Notably, supergroup E was placed at the base of the Wolbachia radiation with maximal statistical support in all analyses ( Fig. 2 ; Supplementary Figs 6–17 ). In none of our analytical approaches a conflicting rooting was proposed. 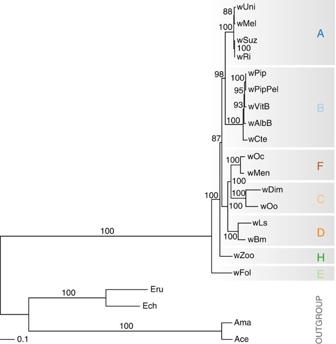Figure 2: Rooted maximum likelihood phylogeny of 21Wolbachiastrains representing all sampled supergroups. The tree was inferred from the complete nucleotide supermatrix and rooted withAnaplasmaandEhrlichiaoutgroups. Bootstrap values from 1,000 replicates are given in percent as numbers on clades. Coloured letters and boxes designate supergroup affiliations forWolbachiastrains. Scale bar corresponds to inferred evolutionary changes. Bayesian inference resulted in the same, maximally supported tree (Supplementary Fig. 7). Furthermore, both Shimodaira–Hasegawa (SH) and approximately unbiased (AU) tests favoured this rooting over any other ( Table 2 ). Consequently, the strain that likely induces parthenogenesis in the collembolan F. candida [25] is the sister group to all other Wolbachia supergroups analysed. Figure 2: Rooted maximum likelihood phylogeny of 21 Wolbachia strains representing all sampled supergroups. The tree was inferred from the complete nucleotide supermatrix and rooted with Anaplasma and Ehrlichia outgroups. Bootstrap values from 1,000 replicates are given in percent as numbers on clades. Coloured letters and boxes designate supergroup affiliations for Wolbachia strains. Scale bar corresponds to inferred evolutionary changes. Bayesian inference resulted in the same, maximally supported tree ( Supplementary Fig. 7 ). Full size image Table 2 Results of Shimodaira–Hasegawa (SH) and approximately unbiased (AU) tests for alternative root positions of the Wolbachia phylogeny. Full size table To control for systematic biases in our phylogenetic reconstructions, we used various approaches, including visual checks for compositional biases via heat maps ( Supplementary Fig. 18 ), data recoding, slow-fast analyses, single-gene analyses, partition jackknifing, exclusion of compositionally biased genes and usage of non-stationary, non-homogenous models (see Methods). None of these analyses demonstrated conflict in our original data set, but instead consistently converged to a single topology ( Figs 1 and 2 ; Supplementary Figs 2–17 ). Insights from shared gene analysis To assess whether the newly proposed groupings are also reflected in shared genes among their genomes, we performed OrthoMCL-clustering using protein sequences of all Wolbachia supergroups. BLAST searches revealed a number of genes being present in all arthropod Wolbachia strains but missing in supergroups C and D ( Supplementary Table 2 ). Most of these genes lack annotation, but two competence-related genes and one phage-related gene could be identified by reciprocal BLAST searches. 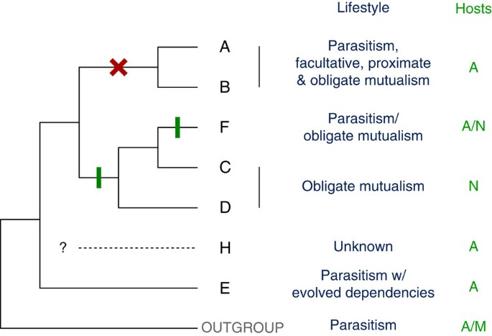Figure 3: Consensus supergroup-levelWolbachiaphylogeny as determined in this study. In blue, lifestyles ofWolbachiasupergroups and the outgroupsAnaplasmaandEhrlichiaare given as defined in ref.34. Hosts are listed in green (A, arthropods; N, nematodes; M, mammals), potential host switches are indicated by green boxes. Notably, only a singleWolbachiaclade (supergroups A and B) can be considered as ubiquitously spread; the ability to adapt to such a broad host range has thus arisen only once (red cross). The placement of supergroup H as inferred in this study remains not fully resolved. In addition, we found that almost all of the 24 phage WO gene products we searched for are present in the assemblies of supergroups E and F ( Supplementary Table 3 ). For phylogenomic analyses of Wolbachia strains, we used a set of 90 informative loci that were recently shown to resolve supergroup level relationships of Wolbachia [16] . We here present a phylogenetic hypothesis of seven Wolbachia supergroups that receives high statistical support throughout all analytical approaches and data sets. Our results suggest that the ability to opportunistically adapt to a large range of hosts has evolved only once in Wolbachia and that major host switches (from arthropods to nematodes or back) have occurred at least twice. This is the most comprehensive phylogenomic analysis of Wolbachia strains to date. Only correct rooting of a phylogeny allows interpreting the directionality of evolutionary events and reconstruction of ancestral states [26] . In some instances, however, distant outgroups may lead to biased reconstructions and long-branch artefacts [27] . Recently, Bordenstein et al . [23] suggested that Wolbachia phylogeny might represent such a case, with closest relatives Anaplasma and Ehrlichia being separated by a comparatively long branch. In the present study, we used multiple approaches to test for systematic biases such as rooting artefacts. The data set was analysed under different nucleotide and amino-acid substitution models (including the CAT model, which suppresses long-branch artefacts [28] ), both with and without outgroups. The impact of compositional biases was explored by visually inspecting compositional heterogeneities via heat maps ( Supplementary Fig. 18 ), using a non-homogeneous, non-stationary nucleotide model of nucleotide sequence evolution and by excluding compositionally biased loci from the amino-acid supermatrix. Furthermore, we reduced the distance between Wolbachia and its outgroups by excluding fast-evolving third-codon positions, by excluding fast-evolving genes, by considering only transversions (in the RY-coded supermatrix) or by recoding amino-acid supermatrices. Confounding effects of potentially recombined genes were assessed with a partition jackknifing approach and with single-gene analyses. Four loci were identified that significantly reject the topology obtained from the complete matrix (SH test, P <0.01), which may be a result of recombination events. However, the topology obtained from a supermatrix without these genes did not differ from the original reconstruction, suggesting that recombination, if present, did not critically bias our results. Finally, SH and AU tests were performed to test for alternative rooting positions. Since none of these approaches suggested the presence of systematic errors or alternative, statistically supported topologies, we conclude that the here presented data and analyses enable the erection of a solid phylogenetic hypothesis for Wolbachia supergroups (consensus in Fig. 3 ). We further infer that the placement of supergroup E at the base of the Wolbachia tree can be considered as robust. Figure 3: Consensus supergroup-level Wolbachia phylogeny as determined in this study. In blue, lifestyles of Wolbachia supergroups and the outgroups Anaplasma and Ehrlichia are given as defined in ref. 34 . Hosts are listed in green (A, arthropods; N, nematodes; M, mammals), potential host switches are indicated by green boxes. Notably, only a single Wolbachia clade (supergroups A and B) can be considered as ubiquitously spread; the ability to adapt to such a broad host range has thus arisen only once (red cross). The placement of supergroup H as inferred in this study remains not fully resolved. Full size image Contrastingly, the placement of supergroup H proved to be not fully resolvable. Depending on the analysis employed, supergroup H was either the sister group of E, sister to all strains except E, sister to (A, B) or sister to (C, F, D). Furthermore, in PhyloBayes analysis the chains did not converge even after >20,000 generations, resulting in an unresolved position of wZoo. Without supergroup H, however, convergence was reached and all splits were highly supported ( Supplementary Fig. 8 ). This inconsistency is very likely due to the limited amount of Wolbachia sequence data recovered from the assembly of wZoo—only 19 of 90 loci could be included in phylogenetic analyses. Since all other splits of the Wolbachia tree received maximal support in almost all approaches used, an increase in loci for wZoo will likely enable a stable placing of this supergroup as well. However, supergoup H was most frequently placed at the base of the tree in our analyses ( Supplementary Figs 2–17 ), either as a sister goup to E or as a sister group to a clade uniting all strains except E. Furthermore, in previous investigations supergroups E and H were consistently recovered as sister groups [8] , [11] , [18] , [23] , [29] , [30] and no conflicting grouping was proposed so far. Consequently, a placement of supergroup H as a sister group to supergroup E has received most support so far and seems most likely, although it could not unequivocally be demonstrated with our analyses ( Fig. 2 ). Several important implications can be deduced from the here presented results. First, the last common ancestor of Wolbachia was likely an endosymbiont of arthropods with a limited host range. Although most obvious in supergroups C and D (which infect only filarial nematodes), a certain degree of host specificity can be observed in all strains except for supergroups A and B ( Fig. 3 ): supergroups E and H are found only in springtails [31] , [32] and termites [29] , respectively, and some supergroup F Wolbachia are also restricted to single host taxa [19] , [33] . Thus, the ubiquitous arthropod Wolbachia that are found in 40% of terrestrial arthropods [2] belong to a single, derived phylogenetic lineage (supergroups A+B). The lifestyle of the last common ancestor of all Wolbachia strains cannot be reconstructed with confidence, as the lifestyles of the two basal branching lineages (supergroups E and H) are not fully understood. Furthermore, Wolbachia lifestyles are not always unambiguous to interpret [34] and the phylogenetic placement of further, potentially distinct Wolbachia lineages is still unclear [23] . However, it has been demonstrated that Wolbachia induces parthenogenesis in F. candida and that in turn F. candida depends on Wolbachia to produce viable offspring [25] , [35] . This argues for some degree of evolved dependency, which is scarcely distributed among arthropod Wolbachia , where CI seems to be the prevailing induced phenotype [3] , [34] . Consequently, supergroups A and B may not only be phylogenetically derived, but also in terms of physiology and thus in impact on their hosts. Comparative genomic analyses especially of basal Wolbachia supergroups could corroborate this hypothesis. Second, our results suggest a sister group relationship between supergroups C and F. This grouping was recovered in a recent analysis using sequences of 52 ribosomal proteins of six Wolbachia strains [36] , as well as in all of our analyses. Since both nematodes and arthropods may carry supergroup F Wolbachia , at least one host switch from nematodes to arthropods (or vice versa) must have occurred within that group ( Fig. 3 ). Some supergroup F Wolbachia act as mutualists in arthropods [13] and in the filarial nematode Mansonella , this strain is essential for the survival of its host, which is similar to what can be observed for supergroups C and D [14] . Moreover, remnants of Wolbachia genes were found in naturally Wolbachia -free filarial nematodes, indicating multiple independent losses of the infection [37] . Therefore, when considering phylogenetic evidence, mutualism may be common in supergroup F and more cases of so far undetected obligate mutualism can be expected in this supergroup. To assess whether supergroup F has emerged only recently in nematodes and thus originated from arthropod hosts [18] , a broader taxon sampling of supergroup F strains is needed. Third, gene content analyses suggest that a number of genes were lost in the genomes of supergroups C and D Wolbachia (see Supplementary Table 2 ). Since the streamlined genomes of these nematode-infecting Wolbachia are a consequence of long-lasting mutualistic relationships with their hosts [38] , [39] , these losses have most likely occurred independently in both lineages. Interestingly, two of the annotated genes present in all arthropod Wolbachia , but missing in supergroups C and D, are competence-related, that is, involved in uptake of external DNA ( Supplementary Table 2 ). Exchange of genetic elements is common in Wolbachia and other endosymbionts [40] , but may be reduced like any other nonessential functions in stable obligate symbioses [41] . Similarly, phage WO genes are absent in supergroups C and D, but might have been present at some time in these groups [42] . Our screen revealed that phage elements are present in all other Wolbachia supergroups (see Supplementary Table 3 ), which is further evidence for convergent secondary losses of phage genes in supergroups C and D. This first comprehensive, rooted phylogeny of the genus Wolbachia shows that supergroups A and B are not only peculiar in the huge diversity of host interactions, their ability to regularly adapt to new hosts and in their pandemic spread, but also that they constitute a phylogenetically derived group within the radiation of Wolbachia strains. Most likely, the bacteria from which Wolbachia originated were less flexible in terms of their host choice. This lifestyle is to some extent reflected in the basal Wolbachia lineages E and H. Alternatively, these basal lineages may be the remnants of a past Wolbachia pandemic that has subsequently been replaced by supergroups A and B, or these lineages have specialized on a single host secondarily. Our results will thus be the basis for further exploring the evolutionary history of Wolbachia . Sampling and sequencing The data sets used in this study were compiled from published Wolbachia genomes (supergroups A, B, C and D), Anaplasma and Ehrlichia outgroups and Wolbachia supergroup F sequence data originating from the Mengenilla moldrzyki sequencing project [43] ( Table 1 ). Furthermore, we performed WGS sequencing of supergroups for which comparable data were so far unpublished or unavailable: supergroup F Wolbachia from O. caerulescens (collected in Fürstenberg/Havel, Germany), supergroup H from Z. nevadensis (collected near Bamfield, BC, Canada), supergroup E from F. candida (kindly provided by David Russell and Ulrich Burkhardt, Görlitz, Germany) and Wolbachia from C. felis (kindly provided by Dieter Striese and Ronny Wolf, Görlitz, Germany and Leipzig, Germany, respectively). DNA was extracted from a single individual of each O. caerulescens (including its Wolbachia strain wOc) and Z. nevadensis (carrying wZoo), and from 10 pooled individuals of F. candida (with wFol) and C. felis (with wCte) by proteinase K digestion and subsequent chloroform extraction. Double-index sequencing libraries with average insert sizes of around 300 bp were prepared as previously described [44] , [45] . The libraries were sequenced as a 125-bp paired-end run on an Illumina Hi-Seq 2000. Raw data processing and assembly Base calling was performed with freeIbis [46] , adapter and primer sequences were clipped and false-paired reads were discarded. We filtered the data by removing all reads that included >5 bases with a quality score below 15. Raw data were submitted to the NCBI sequence read archive under accession numbers SRR1222146 (wZoo), SRR1222150 (wCte), SRR1222159 (wFol) and SRR1221705 (wOc). De novo assemblies were conducted with CLC Genomics Workbench 5.1 (CLC bio, Århus, Denmark) using default settings and with IDBA-UD 1.1.0 (ref. 47 ), using an initial k-mer size of 21, an iteration size of 10 and a maximum k-mer size of 81. For all subsequent analyses, the assemblies with highest N50 values were selected: for wOC, we used the CLC assembly; for wCte, wFol and wZoo, IDBA-UD assemblies were used. Assembly statistics are listed in Supplementary Table 1 . Alignment and phylogenetic analyses In a recent phylogenomic analysis of Wolbachia supergroups A, B, C and D [16] , 90 orthologous loci were identified that meet the following criteria: (1) presence of a single copy in four investigated Wolbachia supergroups and outgroups ( Anaplasma ssp. and Ehrlichia ssp. ), (2) absence of recombination and (3) no evidence for nucleotide substitution saturation. Since these loci were shown to provide a well-resolved supergroup-level Wolbachia phylogeny [16] , we used the same set of orthologues in our analyses. We identified these loci in all assemblies using BLAST+ version 2.2.8 (ref. 48 ). Single loci were translated with TranslatorX version 1.1 (ref. 49 ), aligned with MAFFT version 7.037b [50] using the L-INS-i strategy and then back-translated. Thus we obtained codon-based nucleotide alignments as well as amino-acid alignments. To remove ambiguously aligned positions, we performed alignment masking with Gblocks version 0.91b [51] , allowing small block sizes and gaps (options b4=2 and b5=all). Amino-acid and nucleotide supermatices were constructed with FASconCAT [52] ; best-fitting evolutionary models for these were determined by their BIC (Bayesian information criterion) values with ProtTest version 3.4 (ref. 53 ) and jModelTest version 2.1.3 (ref. 54 ), respectively. We tested for recombination within our data sets using the Pairwise homoplasy index as implemented in PhiPack [55] , with sliding-window sizes of 200, 100, 50 and 25 and 1,000 permutations each. Furthermore, test of nucleotide substitution saturation were performed using Xia’s [56] method, as implemented in DAMBE version 5. Phylogenetic reconstructions of Wolbachia supergroup relationships were conducted with maximum likelihood (ML) methods and Bayesian inference (BI). For the nucleotide supermatrix, a ML tree was inferred with RAxML version 8.0.5 (ref. 57 ) using the model GTR+Γ+I. Branch support was estimated with 1,000 bootstrap replicates. BI was performed with MrBayes version 3.1.2 (ref. 58 ), using GTR+Γ+I. Two times four chains were run for 1 million generations, every 500th generation was sampled. After a deviation of split frequencies of ≤5% was determined, tree information was summarized excluding 250,000 generations as burnin. Posterior probabilities were inferred from clade frequencies of the majority rule consensus tree constructed from the remaining trees. Both BI and ML analyses were separately conducted with identical settings for nucleotide matrices without outgroups. ML analysis of the amino-acid supermatrix was performed with RAxML using the model FLU+Γ+I and calculating bootstrap support from 1,000 replicates. In addition, for BI we employed PhyloBayes MPI version 1.5a (ref. 59 ) with the CAT-GTR model [60] that accounts for substitutional heterogeneities among amino-acid data sets. For all PhyloBayes analyses, two chains with at least 10,000 cycles were run (10,000–24,377; 14,666 on average). All trace parameters were plotted to test whether stationarity had been reached and to diagnose suitable burnin sizes. The chains were stopped after both trees and continuous parameters were diagnosed to have converged with the built-in methods of PhyloBayes (bpcomp & tracecomp). Posterior probabilities were calculated from the clade frequencies of the posterior sample of trees. ML and BI as described above were also conducted for an amino-acid data set without outgroups. For provisional supergroup assignment, we used BLAST+ to search for Wolbachia MLST loci [24] , aligned these with available MLST profiles from Wolbachia PubMLST database ( http://pubmlst.org/wolbachia ) that include a supergroup annotation and performed a ML tree search with RAxML. Assessment of root position and tests for systematic errors To assess the stability of the root position, we calculated 11 separate ML trees with RAxML while enforcing different topologies, each corresponding to a distinct rooting of the Wolbachia ingroup. We then compared the resulting trees with the best tree of the unconstrained ML analysis via a SH-test [61] , as implemented in RAxML. In addition, we calculated per-site log likelihoods for all 12 trees with RAxML and compared the topologies with an AU test using CONSEL version 1.2.0 (ref. 62 ). Both tests were performed with nucleotide and amino-acid supermatrices. Since rooting artefacts may origin from distantly related outgroups [23] , we took recoding and exclusion approaches to reduce the overall evolutionary distances within the data sets and to explore potentially alternative rooting positions. This approach was shown to be suitable to investigate systematic biases in similar data sets [63] . For the nucleotide supermatrix, we performed ML analysis for a RY-coded supermatrix and for a data set without third-codon positions as described above. The amino-acid supermatrix was recoded with the dayhoff6 and dayhoff4 schemes in PhyloBayes. Then, analyses with PhyloBayes were run as described above. Next, we determined pairwise sequence identities (as proxy for evolutionary changes through time) for all loci with the function ‘dist.alignment’ of the R package SequinR [64] . PhyloBayes was then used as described above to infer Wolbachia supergroup phylogeny based on amino-acid matrices without the 20 and 40 fastest-evolving genes. To test for sequence composition biases, we first used BaCoCa Version 1.104r [65] to create descriptive statistics for our amino-acid supermatrix. Taxon to gene-specific heat maps were generated for the proportion of hydrophilic, polar, positively, negatively and neutrally charged amino-acid side chains. These proportions were calculated for all loci and taxa and subject to hierarchical clustering. The resulting heat maps were inspected for conspicuous clusters, especially of Wolbachia strains with outgroups. Heterogeneity in base composition was addressed by employing nhPhyML [66] , which uses a non-homogeneous non-stationary model that accounts for variations in the base composition. Since Wolbachia supergroups were homogeneous in base composition, but the outgroups Anaplasma and Ehrlichia showed pronounced differences ( Supplementary Fig. 14 ), we also performed ML analyses with the nucleotide supermatrix using only Anaplasma and only Ehrlichia outgroups. Because ingroup taxa did not seem compositionally biased, we next identified the loci that significantly deviated from compositional homogeneity and thus potentially skewed our results. To this end, we ran a single chain for 5,000 points with PhyloBayes for each of the 90 loci. Then, we used the implemented test statistics of PhyloBayes (option -comp) to calculate z -scores and P values for compositional deviation. We then excluded all loci with a z -score>2 and a P value<0.05 (33 loci altogether) and reran the PhyloBayes analysis as described above. To further assess what influence single loci have on the topology, we conducted a partition jackknifing approach [67] . Out of 90 loci in total, we randomly picked 30 loci or 60 loci, with 100 permutations each. Then, we analysed each single jackknifed matrix with RAxML. Finally, we counted the number of times each node appeared in the jackknifed analyses as a proxy for the support of that node. Finally, we also analysed single loci with RAxML. We used only the 72 loci that had at least a single representative for all supergroups except supergroup H and removed the taxa for which not all of these 72 loci were available. All single-gene topologies were then summarized to a ‘primordial consensus’ tree using the method by Steel et al . [68] , which accounts for events of potential lateral gene transfers. Gene content analysis To identify genes that might have been lost or gained during Wolbachia’s evolutionary history, we first downloaded the coding sequences of representative Wolbachia strains of supergroups A (wMel, wHa), B (wPip, wNo), C (wOo) and D (wBm) from NCBI. Next, we performed orthologue clustering with OrthoMCL version 2.0 (ref. 69 ) using default settings. We kept the clusters that contained only sequences from supergroups A and B and used them to run BLAST+ searches against the assemblies of wLs (supergroup C) and wDim (supergroup D). We discarded the clusters that returned a significant hit (cutoff at e-value 10E-4) and used the remaining clusters to identify potential orthologues in wFol, wZoo, wOc and wMen with BLAST+. Finally, we ran online BLAST searches on NCBI database to check whether queries and hits were coherently annotated. Furthermore, to gain insights into the evolutionary history of phage acquisition and loss across Wolbachia strains, we searched for gene products of the bacteriophage WO [70] in the assemblies wFol, wZoo, wOc and wMen. How to cite this article: Gerth, M. et al . Phylogenomic analyses uncover origin and spread of the Wolbachia pandemic. Nat. Commun. 5:5117 doi: 10.1038/ncomms6117 (2014). Accession codes: Whole-genome-shotgun data have been deposited in NCBI sequence read archive under BioProject number PRJNA244005 .